Protein encapsulation within synthetic molecular hosts Protein encapsulation has long attracted many chemists and biologists because of its potential to control the structure and functions of proteins, but has been a daunting challenge because of their incommensurably larger size compared with common synthetic hosts. Here we report the encapsulation of a small protein, ubiquitin, within giant coordination cages. The protein was attached to one bidentate ligand and, upon addition of Pd(II) ions (M) and additional ligands (L), M 12 L 24 coordination nanocages self-assembled around the protein. Because of the well-defined host framework, the protein-encapsulated structure could be analysed by NMR spectroscopy, ultracentrifugation and X-ray crystallography. The capture and encapsulation of small guest molecules within synthetic hosts is a vibrant and active field of research focused on controlling the functions, properties and stability of trapped molecules in a manner reminiscent of that of enzymes [1] , [2] , [3] , [4] . Looking beyond small molecules, proteins are naturally occurring giant molecules and tempting targets [5] for encapsulation by synthetic hosts. First, the design and synthesis of a suitable molecular cage for protein encapsulation is a daunting synthetic challenge due to the large size and sensitive nature of proteins. Second, and more importantly, the enclathration of biomolecules will have a significant impact on their chemical properties and should lead to new applications; for example, we envision, as an ultimate goal of this study, that encapsulation could substantially enhance protein stability, alter protein function and facilitate the development of new methods for protein crystallography. In spite of the challenge and potential applications, there have been no reported examples of protein encapsulation by an artificial well-defined molecular host. There are some examples of protein immobilization within polymeric media [6] , [7] , [8] , [9] , [10] , porous solids [11] , [12] and biocapsules (such as proteinaceous capsids [13] , [14] , [15] , [16] and DNA cages [17] ), but these are limited in their applications owing to difficulties in preparation, structure analysis and modification. Only peptide fragments have been recognized by synthetic hosts [18] . Here we report the encapsulation of a small protein, ubiquitin, within giant, self-assembled coordination cages. The protein was attached to one bidentate ligand and, upon addition of Pd(II) ions (M) and additional bidentate ligands (L), M 12 L 24 coordination nanocages self-assembled around the protein. As a consequence of the well-defined host framework, the protein-encapsulated structure could be well analysed by NMR spectroscopy, ultracentrifugation and X-ray crystallography coupled with the maximum-entropy method (MEM) that clearly mapped the electron density of the protein in the coordination cage. We expect that protein encapsulation by the cages will allow us to explore the function [19] , [20] of synthetic hosts for the conformational and functional control of encapsulated proteins. Design and synthesis of protein-encapsulating cages Unlike most synthetic hosts, our giant M 12 L 24 coordination spheres [21] , [22] , [23] , self-assembled from 12 Pd(II) ions (M) and 24 bent ligands (L), display nanometer-sized cavities that can be expanded up to 7.3 nm in diameter, simply by lengthening the ligand arms. With giant coordination spheres in hand, we set our sights on the enclathration of proteins. As our first target, we choose ubiquitin, a relatively small globular protein (76 residues, 8.6 kDa, approximately 3–4 nm in diameter) that has an important role in proteasomal degradation [24] , [25] . In our strategy, ubiquitin is covalently attached to the interior edge of one of the 24 ligands of the M 12 L 24 sphere framework ( Fig. 1a ). As modification of the carboxy terminus of ubiquitin does not affect the protein structure, the Gly76 residue at the carboxy terminus was mutated to Cys to facilitate the covalent attachment to the N -substituted maleimide of ligand 4 . By treating the Gly-to-Cys mutant of ubiquitin with excess 4 , we obtained the ubiquitin ligand 2a in >60% overall yield ( Fig. 1b ) [26] . 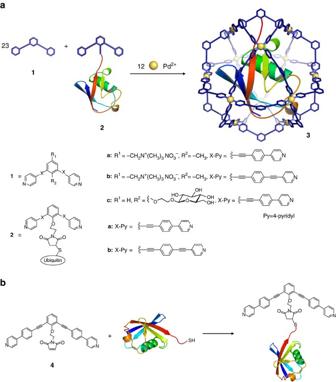Figure 1: Schematic representation of the encapsulation of ubiquitin. (a) Self-assembly of ubiquitin-containing spheres3. Ubiquitin was encapsulated within3by assembly of ligand1around ubiquitin ligand2upon addition of Pd(II) ions at 45 °C for 3 h. (b) Preparation of ubiquitin-attached ligand2afrom4aand Gly76Cys-mutated ubiquitin25. Figure 1: Schematic representation of the encapsulation of ubiquitin. ( a ) Self-assembly of ubiquitin-containing spheres 3 . Ubiquitin was encapsulated within 3 by assembly of ligand 1 around ubiquitin ligand 2 upon addition of Pd(II) ions at 45 °C for 3 h. ( b ) Preparation of ubiquitin-attached ligand 2a from 4a and Gly76Cys-mutated ubiquitin [25] . Full size image With ligand 2a , we examined the self-assembly of ubiquitin-containing mixed M 12 L 24 spheres ( Fig. 1a ). The large size of ubiquitin (3–4 nm) prohibits the encapsulation of multiple proteins, and thus, equilibrium among all the components (the metals and ligands) should favour the assembly of spheres containing only one ubiquitin molecule. The tertiary structure of ubiquitin is retained in aqueous solution, as indicated by the amide protons in the 1 H and 1 H- 15 N heteronuclear single-quantum coherence NMR spectra [26] , and ligand 1a with its apical Me 3 N + moiety was chosen for sphere formation due to its increased solubility in the aqueous solvent mixture. Ubiquitin ligand 2a was treated with ligand 1a (30 equiv) and Pd(NO 3 ) 2 (17 equiv) in D 2 O/CD 3 CN (1:1) at 45 °C for 3 h, and characteristically simple 1 H NMR spectra indicated the quantitative self-assembly of coordination spheres; the pyridine α-proton signals shifted downfield (Δ δ =0.48 ppm) upon coordination of Pd 2+ ( Fig. 2 ). 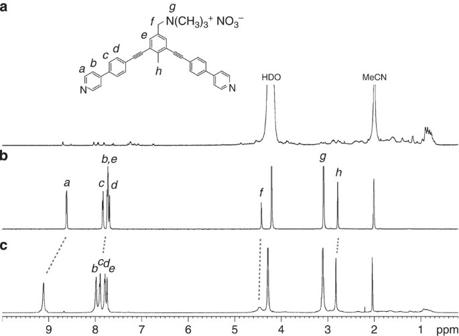Figure 2:1H NMR spectra of the encapsulation of ubiquitin within coordination spheres. (a) Ubiquitin ligand2a. (b) Ligand1a. (c) Ubiquitin-containing sphere3aafter treating ubiquitin ligand2awith ligand1a(30 equiv) and Pd(NO3)2(17 equiv) in D2O/CD3CN (1:1, 0.5 ml) at 45 °C for 3 h. Downfield shifts of the signals of the pyridine rings (Ha, Hb) confirm the formation of Pd-pyridine bonds in coordination sphere3a, and the simple spectrum indicates the quantitative self-assembly of ubiquitin-containing sphere3a. All spectra recorded at 500 MHz, in D2O:CD3CN=1:1, at 300 K. Figure 2: 1 H NMR spectra of the encapsulation of ubiquitin within coordination spheres. ( a ) Ubiquitin ligand 2a . ( b ) Ligand 1a . ( c ) Ubiquitin-containing sphere 3a after treating ubiquitin ligand 2a with ligand 1a (30 equiv) and Pd(NO 3 ) 2 (17 equiv) in D 2 O/CD 3 CN (1:1, 0.5 ml) at 45 °C for 3 h. Downfield shifts of the signals of the pyridine rings (H a , H b ) confirm the formation of Pd-pyridine bonds in coordination sphere 3a , and the simple spectrum indicates the quantitative self-assembly of ubiquitin-containing sphere 3a . All spectra recorded at 500 MHz, in D 2 O:CD 3 CN=1:1, at 300 K. Full size image Characterization by diffusion-ordered NMR spectroscopy Analysis by diffusion-ordered NMR spectroscopy (DOSY) confirmed the presence of the giant coordination sphere; the diffusion coefficient D of ligand 1a , 3.4×10 −10 m 2 s −1 , log D =–9.47, decreased in magnitude upon complex formation, 7.6×10 −11 m 2 s −1 , log D =–10.12 ( Fig. 3b ), and is identical to that of similar, but empty M 12 L 24 spheres ( Fig. 3d ) assembled from 1a and related analogues. More importantly, the diffusion coefficient of the ubiquitin signals (ranging from 1–6 ppm) also slowed from 1.2×10 −10 (log D =–9.92) to 7.6×10 −11 m 2 s −1 (log D =–10.12), which demonstrates that ubiquitin (roughly 4 nm in diameter) was fully encapsulated within the 6.3 nm coordination sphere 3a . 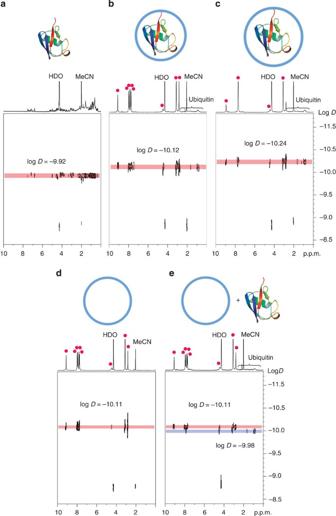Figure 3:1H DOSY NMR spectra of ubiquitin, ubiquitin-containing spheres and empty speheres. Spectra of (a) free ubiquitin (logD=–9.92), (b) ubiquitin-containing sphere3a(logD=–10.12) and (c) ubiquitin-containing sphere3b(logD=–10.24). The diffusion coefficients (D) of ubiquitin significantly decreased and were observed at the sameDvalue as those of sphere3aand3b, respectively, which confirms the encapsulation of ubiquitin within the hollow coordination spheres. Spectra of (d) empty sphere5aand (e) a mixture of free ubiquitin and empty sphere5a. The differentDvalue for ubiquitin and empty sphere5aclearly shows that the simple mixing of ubiquitin and the coordination sphere did not result in the inclusion complex.1H signals of the cage framework of the coordination spheres are marked with red circles. All spectra recorded at 500 MHz, in D2O:CD3CN=1:1, at 300 K. Figure 3: 1 H DOSY NMR spectra of ubiquitin, ubiquitin-containing spheres and empty speheres. Spectra of ( a ) free ubiquitin (log D =–9.92), ( b ) ubiquitin-containing sphere 3a (log D =–10.12) and ( c ) ubiquitin-containing sphere 3b (log D =–10.24). The diffusion coefficients ( D ) of ubiquitin significantly decreased and were observed at the same D value as those of sphere 3a and 3b , respectively, which confirms the encapsulation of ubiquitin within the hollow coordination spheres. Spectra of ( d ) empty sphere 5a and ( e ) a mixture of free ubiquitin and empty sphere 5a . The different D value for ubiquitin and empty sphere 5a clearly shows that the simple mixing of ubiquitin and the coordination sphere did not result in the inclusion complex. 1 H signals of the cage framework of the coordination spheres are marked with red circles. All spectra recorded at 500 MHz, in D 2 O:CD 3 CN=1:1, at 300 K. Full size image Increasing the diameter of the self-assembled coordination sphere further slowed the diffusion of ubiquitin, as indicated by the log D value. Simple insertion of a second acetylene spacer into the backbone of ligand 1b increased the diameter of the coordination sphere to 7.3 nm, and concomitantly, the D value of the nanosphere decreased from 7.6×10 −11 (log D =–10.12, 3a ) to 5.7×10 −11 m 2 s −1 (log D =–10.24, 3b ; Fig. 3c ). Again, the diffusion coefficients for the ubiquitin signals were reduced to an identical value of log D . When ubiquitin was added to a solution containing empty coordination sphere 5a (which was prepared from 12 Pd(NO 3 ) 2 and 24 ligand 1a ), the diffusion coefficient of ubiquitin and sphere 5a remained distinctly different ( Fig. 3d,e ); D =1.0×10 −10 m 2 s −1 , log D =–9.98 and D =7.8×10 −11 m 2 s −1 , log D =–10.11, respectively, and clearly indicate that encapsulation is necessary for the diffusion constant of ubiquitin to decrease to that of the larger nanosphere. Thus, the coincident D values for the 1 H signals of ubiquitin and the cage framework of 3a , b arise from ubiquitin encapsulated within the coordination spheres. Characterization by analytical ultracentrifugation The analytical ultracentrifugation (AUC) experiments confirmed the quantitative formation of ubiquitin-containing sphere 3a . AUC sedimentation velocity measurements ( Fig. 4a ) clearly showed the high monodispersity of 3a in solution, distinguishable from that of empty sphere 5a . More importantly, weight average molecular weights ( M w ) of 3a and 5a were determined from AUC sedimentation equilibrium analyses, employing experimentally estimated partial specific volume ( Fig. 4b ), as 26,300 and 16,300, respectively, in good agreement with their theoretical values of 25,300 and 16,700. 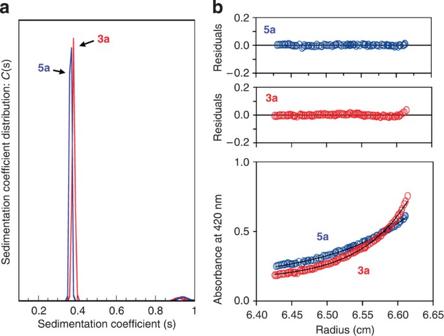Figure 4: Analytical ultracentrifugation experiments. Analytical ultracentrifugation (AUC) results of the vacant sphere5aand the ubiquitin-containing sphere3aat loading concentrations of 2 mM. (a) Plot of the distribution of sedimentation coefficients (C(s) versus s, where s is plotted in Svedberg units, S) calculated from AUC sedimentation velocity experiments. The sharp single peak shows the highly monodisperse nature of5aand3a, and demonstrates the exclusive formation of3a. (b) Concentration gradient of AUC sedimentation equilibrium experiments at 40,000 r.p.m. By non-linear fittings, weight average molecular weights (Mw) were determined as 16,300 for5aand 26,300 for3a, which are in good agreement with their calculated molecular weights: 16,700 for5aand 25,300 for3a. Random distributions of residuals for the non-linear fitting using single species model indicate well fit of the equilibrium concentration gradients. Figure 4: Analytical ultracentrifugation experiments. Analytical ultracentrifugation (AUC) results of the vacant sphere 5a and the ubiquitin-containing sphere 3a at loading concentrations of 2 mM. ( a ) Plot of the distribution of sedimentation coefficients ( C (s) versus s, where s is plotted in Svedberg units, S) calculated from AUC sedimentation velocity experiments. The sharp single peak shows the highly monodisperse nature of 5a and 3a , and demonstrates the exclusive formation of 3a . ( b ) Concentration gradient of AUC sedimentation equilibrium experiments at 40,000 r.p.m. By non-linear fittings, weight average molecular weights ( M w ) were determined as 16,300 for 5a and 26,300 for 3a , which are in good agreement with their calculated molecular weights: 16,700 for 5a and 25,300 for 3a . Random distributions of residuals for the non-linear fitting using single species model indicate well fit of the equilibrium concentration gradients. Full size image Crystallographic analysis of the protein-encapsulating cage To unambiguously confirm the ubiquitin-containing structure of 3 , we concentrated on the crystallographic analysis of the cage. Our earlier attempts to crystallize 3a , b were unsuccessful, most likely because of the high mobility of the dangling ubiquitin molecule in the cage. To appropriately fill the void in the cage and reduce the tumbling motion of the protein, we designed the new sugar-functionalized ligand 1c . The sugar pendant is considered the most suitable for the interior fictionalization, because the hydrophilic molecules can mildly wrap the protein without denaturing its native structure (see Supplementary Fig. S3 for molecular modelling). The ubiquitin-containing cage 3c was prepared from 1c and 2a in a similar manner to 3a , b , and its formation was confirmed by DOSY NMR spectroscopy ( Supplementary Fig. S10 ). X-ray quality single crystals were obtained by slow diffusion of isopropyl acetate vapour into a dimethyl sulfoxide (DMSO) solution of 3c (BF 4 salt; inset of Fig. 5c ). The presence of ubiquitin in the crystals of 3c was confirmed by SDS–PAGE analysis ( Supplementary Fig. S4 ), which was performed after dissolving the crystals in DMSO. By optimizing the crystal quality and the sampling method, and by using a macromolecular crystallography beamline (BL38B1 at SPring-8), considerably high-quality diffraction data up to 1.8 Å resolution were collected. 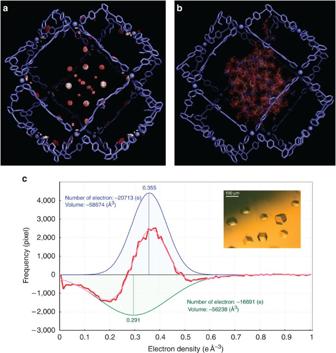Figure 5: MEM refinement of the structure of3c. (a) The crystal structure of3c. Only the M12L24spherical shell was modelled by conventional crystallographic analysis. Within the3cshell, the MEM-refined electron density ascribable to ubiquitin was mapped (red: 0.35 eÅ−3, a value determined by electron density histogram analysis; white: 0.39 eÅ−3, a typical electron density of protein). (b) The combination of the crystal structure of3cand the modelling of a ubiquitin molecule. (c) The difference in the electron density histogram between ubiquitin-containing sphere3cand empty sphere5cis shown. A positive narrow peak at 0.35 eÅ−3(blue) and a negative broad peak at around 0.29 eÅ−3(green) are observed. The positive peak is close to the typical electron density of proteins (0.39 eÅ−3) and thus attributed to the ubiquitin electron density. The negative peak is consistent with the value of 0.29–0.35 eÅ−3for the DMSO–isopropyl acetate mixed solvent. Thus, the histogram difference clearly shows the presence of ubiquitin and the exclusion of solvents in the void of3c. For further details, seeSupporting Online Materials. Inset: a picture of the crystals of3c. Figure 5: MEM refinement of the structure of 3c . ( a ) The crystal structure of 3c . Only the M 12 L 24 spherical shell was modelled by conventional crystallographic analysis. Within the 3c shell, the MEM-refined electron density ascribable to ubiquitin was mapped (red: 0.35 eÅ −3 , a value determined by electron density histogram analysis; white: 0.39 eÅ −3 , a typical electron density of protein). ( b ) The combination of the crystal structure of 3c and the modelling of a ubiquitin molecule. ( c ) The difference in the electron density histogram between ubiquitin-containing sphere 3c and empty sphere 5c is shown. A positive narrow peak at 0.35 eÅ −3 (blue) and a negative broad peak at around 0.29 eÅ −3 (green) are observed. The positive peak is close to the typical electron density of proteins (0.39 eÅ −3 ) and thus attributed to the ubiquitin electron density. The negative peak is consistent with the value of 0.29–0.35 eÅ −3 for the DMSO–isopropyl acetate mixed solvent. Thus, the histogram difference clearly shows the presence of ubiquitin and the exclusion of solvents in the void of 3c . For further details, see Supporting Online Materials . Inset: a picture of the crystals of 3c . Full size image The crystal structure analysed using conventional crystallographic methods clearly showed the roughly spherical M 12 L 24 framework of 3c within a huge cell volume of 195,900 Å 3 . The cavity volume of the sphere itself is estimated to be 63,500 Å 3 , large enough to accommodate ubiquitin. However, we could not build a structural model of ubiquitin by conventional structure analysis due to the intrinsic orientational disorder of the ubiquitin moiety in the highly symmetric M 12 L 24 framework. In the electron density map, only hazy residual electron density was observed, and this could not be used for the structural elucidation of the encapsulated ubiquitin. To refine the electron density, the MEM [27] , [28] , [29] , [30] was applied, which is a powerful information-processing method that allows us to obtain more precise electron density even from limited data with low resolution and errors. After applying the MEM, the electron density ascribable to ubiquitin (0.39 eÅ −3 , a typical electron density of proteins) was mapped in the crystal structure ( Fig. 5a ). The three-dimensional distribution of the 0.39 eÅ −3 electron density matched quite well to the geometrical arrangement of the ubiquitin moiety in the optimized structure of 3c ( Fig. 5b ). We thus conclude that the localized electron distribution of ubiquitin was clearly uncovered inside the cage, proving the encapsulation of ubiquitin in the synthetic host. The electron density after the MEM refinement was further analysed quantitatively. The red line in Fig. 5c shows the difference between the electron density histograms of ubiquitin-containing sphere 3c and empty sphere 5c . This histogram difference was fitted with one positive and one negative Gaussian curve (blue and green lines) by the least-squares method: a clear narrow positive peak at 0.35 eÅ −3 , close to the average electron density of proteins (typically, 0.39 eÅ −3 ), and a broadened negative peak centred at around 0.29 eÅ −3 , close to the value of 0.29–0.35 eÅ −3 for DMSO–isopropyl acetate mixed solvent. The real-space volumes corresponding to the positive and negative regions are about 59,000 and 56,000 Å 3 , respectively, which are roughly equal to the volume of a 40 Å diameter sphere that can fully include ubiquitin. Thus, the histogram difference clearly shows the inclusion of ubiquitin and the exclusion of solvents in the void of 3c . The first encapsulation of a protein within synthetic host molecules reported here marks an important milestone. We succeeded in utilizing self-assembly to construct cage frameworks around a covalently tethered protein, and the synthetic accessibility and modular nature of our coordination spheres promises a useful range of host cages for the encapsulation of proteins and enzymes of various sizes and shapes. There are some examples of protein immobilization within synthetic media (polymers [6] , [7] , [8] , [9] , [10] and porous solids [11] , [12] ). Our discrete cage host however makes a clear distinction from these ill-defined host media in that the encapsulated proteins can be easily addressed by conventional powerful analysis tools. All the analysis methods employed here, including DOSY NMR, AUC, SDS–PAGE analysis ( Supplementary Fig. S4 ), and X-ray crystallography coupled with MEM analysis, are not applicable to the characterization of previous hosts, thus providing the reliable and direct characterization of the protein-encapsulated host. More importantly, this great advantage over the previous methods makes possible the precise design of the structure and functions of proteins. In terms of application, the protein encapsulation by synthetic discrete hosts is a long-term project and in the present study, we addressed the initial synthetic challenge. We believe this work lays the foundation for further steps towards our ultimate goal of utilizing coordination cages for the conformational and functional control of encapsulated proteins [19] , [20] . General NMR spectra were obtained on a Bruker DRX-500 spectrometer equipped with a 5 mm BBO Z -gradient probe, on a Bruker AV-500 equipped with TCI gradient CryoProbe, or on a JEOL ECA-600 equipped with gradient cold probe (53040HCNVC). The chemical shift values reported here are with respect to an internal tetramethylsilane (TMS) standard. MALDI-TOF (matrix-assisted laser/desorption ionization time-of-flight) mass spectra were measured with a TOF mass spectrometer (Applied Biosystem Voyager DE-STR) equipped with a MALDI source. Cold-spray ionization-TOF mass and high-resolution electrospray ionization-TOF mass spectra were measured on a Bruker maXis. The data analyses of mass spectra were processed on a Bruker DataAnalysis (Version 4.0 SP 2) software and the simulations were performed on a Bruker IsotopePattern software. Infrared (IR) measurements were carried out as KBr pellets using a DIGILAB Scimitar FTS-7000 instrument. Melting points were determined on a Yanaco MP-500 V melting-point apparatus. Elemental analyses were performed on a Yanaco MT-6. Solvents and reagents were purchased from TCI Co., Ltd., WAKO Pure Chemical Industries Ltd. and Sigma-Aldrich Co. All the chemicals were of reagent grade and used without any further purification. Self-assembly of sphere 3c Ligand 1c (0.77 mg, 1.2 μmol) and ubiquitin ligand 2a (0.36 mg, 0.04 μmol) were treated with [Pd(MeCN) 4 ](BF 4 ) 2 (0.43 mg, 0.97 μmol) in DMSO- d 6 (0.25 ml) at 50 °C for 1.5 h. The formation of the ubiquitin-including sphere 3c was confirmed by 1 H NMR and 1 H DOSY NMR spectroscopy; 1 H NMR (500 MHz, DMSO- d 6 , 300 K) δ 9.33 (br, 96H), 8.17 (br, 96H), 7.96 (br, 96H), 7.76 (br, 96H), 7.60 (br, 48H), 7.23 (br, 24H), 4.98 (br, 48H), 4.88 (br, 24H), 4.51 (br, 48H), 4.46 (br, 24H), 4.29 (d, J =7.6 Hz, 24H), 4.24 (br, 24H), 3.99 (br, 24H), 3.66 (br, 24H), 3.46 (br, 24H), 3.17 (br, 24H), 3.11 (br, 48H), 3.06 (br, 24H). Broad signals of ubiquitin were observed at 0.7–3 ppm. Diffusion coefficient D =3.2×10 −11 m 2 s −1 (DMSO- d 6 , 300 K) from 1 H nuclei. Spheres 3a and 3b were prepared in a similar way. Analytical ultracentrifugation AUC sedimentation velocity (AUC-SV) and sedimentation equilibrium (AUC-SE) experiments were performed in DMSO containing 30 mM calcium nitrate, using Proteomelab XL-I Analytical Ultracentrifuge (Beckman-Coulter). In AUC-SV analysis, 2 mM samples of M 12 L 24 sphere and ubiquitin-containing mixed M 12 L 24 sphere were measured. Runs were carried out at 60,000 r.p.m. and at a temperature of 20.0 °C using 12 mm charcoal-epon double sector centerpieces and An60 Ti analytical rotor. The evolution of the resulting concentration gradient was monitored with absorbance detection optics at 390 nm, All AUC-SV raw data were analysed by the continuous C (s) distribution model in the programme SEDFIT11.71 (ref. 31 ). As for AUC-SE analysis, samples at different loading concentrations between 0.25 and 4 mM were examined. Runs were carried out at 40,000 r.p.m. and at a temperature of 20.0 °C using 12 mm charcoal-epon double sector or six-channel centerpieces, and An50 Ti or An60 Ti analytical rotors. The equilibrium concentration gradient was monitored at 390, 420 or 425 nm according to sample concentrations. All AUC-SE data were analysed by using the programme Origin 6.0 (Originlab Corporation). Partial specific volume of 5a was experimentally determined as 0.7098 cm 3 g −1 from density measurement of sample solutions with different concentrations using DMA5000 (Anton Paar, Graz, Austria) [32] . Partial specific volume of 3a was estimated as 0.7182 cm 3 g −1 according to values of M 12 L 24 sphere and ubiquitin with the assumption that one ubiquitin molecule is encapsulated in one M 12 L 24 sphere. The density and viscosity of DMSO used for the analysis was 1.10022 g cm −3 and 1.996 centipoises, respectively. Preparation of single crystals of 3c Crystals of 3c for X-ray diffraction analysis were obtained by vapour diffusion of isopropyl acetate into a 0.42 mM DMSO solution of 3c at 20 °C. 3c crystallized after the solution volume was roughly doubled. X-ray diffraction data was collected using high-flux and low-divergence synchrotron X-ray irradiation. The crystals were mounted on a goniometer and cooled to 100 K in a N 2 cryostream as quickly as possible, to avoid the degradation in crystal quality. As cryoprotectants severely damage the crystal, the data were collected without them. Data collection and MEM analysis The diffraction data were collected at BL38B1 in SPring-8 (Sayo, Hyogo, Japan). The structure determination of cage 3c and 5c was performed by molecular replacement followed by MEM analysis with the programme ENIGMA [33] . The crystal data are summarized in Supplementary Information . To perform MEM analysis, the total number of electrons in the unit cell must be estimated. The average electron density in the solvent is estimated to 0.32 eÅ −3 , as the solvent is composed of an equimolar ratio of DMSO and isopropyl acetate, the average electron density of which are 0.35 and 0.29 eÅ −3 , respectively. The total number of electrons in the non-ubiquitin- and ubiquitin-encapsulated structures are calculated to be 68,500 and 70,000, respectively. For comparison, the non-ubiquitin structure was also analysed. The collected diffraction data were processed by HKL2000 (ref. 34 ). The structure was solved by molecular replacement with MOLREP (ref. 35 ) using empty M 12 L 24 ( 5c ) model and was refined with SHELXL97 (refs 36 , 37 ). The total number of electrons TE of 5c crystal for MEM analysis is given by the following equation: TE 5c =the volume of unit cell (≈196,000 Å 3 ) × the fraction of solvent area (≈0.9) × the average electron density of solvent (≈0.32 eÅ −3 ) + the number of electrons of M 12 L 24 (≈6,000) × the number of M 12 L 24 in unit cell (=2). The fraction of solvent area is calculated by MATTHEWS, in which the molecular mass of M 12 L 24 is about 11.5 kDa. The total number of electrons TE 3c of 3c crystal is also given by the following equation: TE 3c = TE 5c + the volume of ubiquitin (≈10,000 Å 3 ) × (the average electron density of ubiquitin (≈0.39 eÅ −3 ) − the average electron density of solvent (≈0.32 eÅ −3 )) × the number of ubiquitin in unit cell (=2). The average electron density of ubiquitin is obtained by dividing the total electron, 3,926, by the volume. The space-group of 3c crystal was determined by extinction rule and self-rotation function calculated preliminarily in P 1 with MOLREP, in which the cut-off radius was set at the length of M 12 L 24 molecular vector, 51 Å ( Supplementary Fig. S2 ). The space-group symmetry of vacant M 12 L 24 ( 5c ) crystal, I m3¯ m, was reduced to I 222, to compare the density distribution and the histogram with 3c crystal. Synthesis and compound characterization Synthesis and characterization of ligands 1a , 1b , 1c , 2a and 2b are described in Supplementary Information . How to cite this article: Fujita, D. et al . Protein encapsulation within synthetic molecular hosts. Nat. Commun. 3:1093 doi: 10.1038/ncomms2093 (2012).